Horizontal gene transfer of a vertebrate vasodilatory hormone into ticks The horizontal gene transfer (HGT) of functional molecules is found in higher eukaryotes, but its influence on their evolution has not been fully evaluated. Here we describe the HGT of a vertebrate vasodilator, adrenomedullin (ADM), into ticks of the genus Ornithodoros and hypothesize its involvement in tick evolution. The salivary glands of Ornithodoros ticks contain ADM-like vasodilators, tick-adrenomedullin (TAM). ADM-like molecules, including TAM, are conserved in all vertebrates and Ornithodoros ticks but not in any other invertebrates, including Argas ticks, which share a common ancestor with Ornithodoros ticks. In addition, the close evolutionarily relationship between TAM and ADM is supported through genomic sequence and phylogenetic relatedness analyses. Ornithodoros ticks horizontally acquired vertebrate ADM and currently employ it to facilitate blood feeding. The acquisition of TAM might result in a beneficial change in feeding behaviour and influence the divergence of Ornithodoros ticks. Horizontal gene transfer (HGT) refers to the movement of genetic information between distantly related organisms. In prokaryotes, the HGT of functional molecules has contributed to their antibiotic resistance and virulence, and HGT is widely recognized as an important evolutionary force [1] . In higher eukaryotes, the HGT of functional molecules has also been demonstrated [2] , [3] , [4] . However, its frequency is decreased in higher eukaryotes compared with prokaryotes because the transmitted genes must be introduced into germ-line cells [5] . Even transmitted genes that are successfully integrated into the genome of germ-line cells are not necessarily transcribed in the recipient cells and could thus become pseudogenized [6] , [7] , [8] . Therefore, only a few examples have demonstrated that horizontally transmitted molecules actually influence the biology of recipient cells in higher eukaryotes, and the role of the HGT of functional molecules has not yet been fully evaluated in their evolution. Adrenomedullin (ADM) is a peptide hormone that originated in an ancestral vertebrate, perhaps a cyclostome, and is widely conserved among all extant vertebrates [9] . This peptide hormone exhibits various physiological activities, such as hypotensive and angiogenic effects [10] . In particular, it exhibits strong vasodilatory (that is, blood pressure-lowering) activity by directly affecting vascular endothelial cells and smooth muscle cells [11] . ADM can be classified into three major isoforms: ADM-1, ADM-2 and ADM-5 (ref. 12 ). The minor isoforms, ADM-4 and -3, are presumed to have resulted from the gene duplication of ADM-1 and -2, respectively, and are found exclusively in fish [12] . ADM-1 and -2 are widely conserved in all vertebrates. However, ADM-5 is conserved in fish, amphibians and reptiles but has been lost in birds and many mammals, for example, humans, chimpanzees, rats and mice [13] , due to the loss of functional constraints. ADM-1, -2 and -5 are all expressed as pre-proproteins and contain secretory signal peptides and internal processing sites. ADM-1 precursors uniquely include another vasodilatory peptide hormone, proadrenomedullin N-terminal 20 peptide, known as PAMP [14] . All mature ADM isoforms contain a ring-shaped structure consisting of six amino acids; the ring is formed through disulphide bonds between conserved Cys residues. In addition, all of them have an amidated Tyr residue in the C terminus. These Cys residues and modified C-terminal residue are essential for the vasodilatory activities of ADM [15] . Ticks are ectoparasites, and their saliva contains various bioactive molecules that are injected into the body of the vertebrate host during feeding. These molecules facilitate blood feeding by inhibiting host biological defenses, such as blood clotting, platelet aggregation, immune responses and vasoconstriction [16] , [17] . Recently, transcriptomic and proteomic analyses of salivary gland molecules of two Argasidae family ticks, Ornithodoros parkeri and O. coriaceus , have revealed a large number of novel candidate bioactive molecules [18] , [19] , [20] . Interestingly, molecules that resemble vertebrate ADM were found among these candidates, suggesting that the genes may be horizontally transferred from vertebrates. However, no further investigations regarding their function and phylogenetic relationships have been performed, and thus the origin of these molecules remains unclear. Here we identify an ADM-like molecule, designated tick-adrenomedullin (TAM), from the salivary glands of O. moubata , a tick belonging to the family Argasidae . TAM exhibits strong vasodilatory activity in vertebrate hosts. Subsequent genomic sequence analyses of TAM and vertebrate ADMs show exon similarities, suggesting their close evolutionary relatedness. Therefore, these results suggest that Ornithodoros ticks acquired exons encoding the ADM gene horizontally from vertebrate hosts. Currently, Ornithodoros ticks employ this horizontally transmitted hormone to facilitate blood feeding from hosts. Identification of a novel vasodilator TAM To identify novel bioactive molecules in tick salivary glands, we constructed a cDNA library from the salivary glands of O. moubata and then conducted sequence analyses of 1,000 randomly selected clones. Among the analysed clones, 460 cDNA clones encoded putative secretory proteins containing signal peptide sequences ( Supplementary Fig. 1 and Supplementary Data 1 ). As bioactive molecules are secreted into the saliva after intracellular synthesis, these O. moubata cDNA clones were predicted to encode bioactive molecules. These bioactive molecule candidates were further classified into the following six protein families: lipocalin, Kunitz-type protease inhibitor, salivary basic tail-less protein, putative salivary protein type-1, putative salivary protein type-2 and vertebrate ADM-like molecules, that is, TAM ( Supplementary Data 1 ). The TAM family clones found in O. moubata consisted of three different isoforms, designated TAM-a, -b and -c ( Supplementary Fig. 2 ). Similar molecules were discovered in other Ornithodoros ticks, O. parkeri and O. coriaceus , as previously described ( Supplementary Fig. 2 ) [18] , [19] . All of the identified TAM isoforms contained unique amino acid sequence motifs conserved among the major isoforms of vertebrate ADMs ( Fig. 1 ). TAM isoforms contain two Cys residues that are fully conserved among all vertebrate ADM isoforms ( Fig. 1 ). Additionally, all TAM isoforms possessed two putative processing sites that are conserved in ADM-1 and -5. ADM-2 has the N-terminal processing site but completely lacks the C-terminal processing site ( Fig. 1 ). All TAM isoform precursors lacked the region corresponding to PAMP, suggesting no additional peptide hormones similar to PAMP. Vertebrate ADMs generally have an amidated Tyr residue at their C termini [11] ; similarly, the C-terminal residues of mature TAM-a and -b were predicted to be Tyr residues that were expected to be amidated ( Supplementary Fig. 2 ). Conversely, mature TAM-c was predicted to have a Pro as its C-terminal residue ( Supplementary Fig. 2 ). This Pro may also be amidated given that thyrocalcitonin, a peptide hormone in the same protein family as ADM (the calcitonin gene-related peptide family), has an amidated Pro residue at its C terminus [21] . Therefore, based on these structural similarities between TAM and vertebrate ADMs, we assumed that TAM is synthesized as a pre-proprotein in tick salivary gland cells and that it is then post-translationally modified in the same manner as vertebrate ADM, including cleavage by a protease and amidation of the C-terminal residues to form the mature, bioactive molecule. 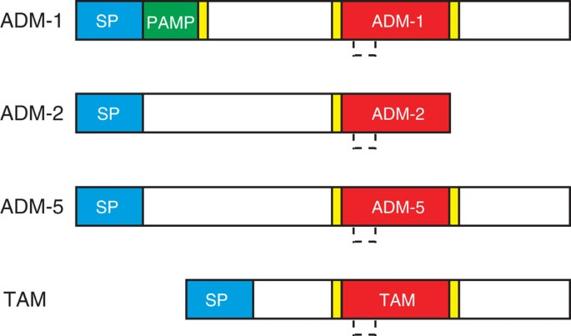Figure 1: Schematic representation of TAM and three major isoforms of vertebrate ADMs, ADM-1, -2 and -5. Blue indicates the signal peptide (SP) sequences, and red indicates regions comprising mature ADM molecules, including TAM. Yellow indicates the processing sites used to liberate mature vertebrate ADM and PAMP. The putative TAM-processing sites are also shown in yellow. The two conserved Cys residues are indicated by dashed lines. Figure 1: Schematic representation of TAM and three major isoforms of vertebrate ADMs, ADM-1, -2 and -5. Blue indicates the signal peptide (SP) sequences, and red indicates regions comprising mature ADM molecules, including TAM. Yellow indicates the processing sites used to liberate mature vertebrate ADM and PAMP. The putative TAM-processing sites are also shown in yellow. The two conserved Cys residues are indicated by dashed lines. Full size image Next, to examine TAM vasodilatory activity, we chemically synthesized the predicted mature form of TAM-a, designated sTAM-a ( Fig. 2a ), and examined its blood pressure-lowering activity. As amidation of the C-terminal residue and formation of disulphide bonds between conserved Cys residues are essential for vertebrate ADM activity [15] , we synthesized TAM-a with these modifications. Eventually, sTAM-a was obtained with a purity of 99.3%. In rats, the intravenous administration of 200 or 500 pmol kg −1 of sTAM-a resulted in a marked decrease in blood pressure ( Supplementary Fig. 3 ). This result suggested that the disulphide bonds between conserved Cys residues and amidated C-terminal Tyr residue are essential for the vasodilatory activity of TAM and that the TAM molecule precursors would be cleaved at both putative processing sites. In contrast, when rat ADM-1 was administered at the same doses, its blood pressure-lowering activity was weaker than that of sTAM-a ( Supplementary Fig. 3 ). Furthermore, a comparison of the concentration-dependent blood pressure-lowering activity of sTAM-a with that of rat ADM-1 clearly showed that sTAM-a possessed a blood pressure-lowering activity 10 times greater than that of rat ADM-1 ( Fig. 2b ). These results demonstrated that TAM-a functions as a vasodilatory hormone in host animals and suggested that O. moubata ticks utilize TAM hormones to facilitate blood feeding. 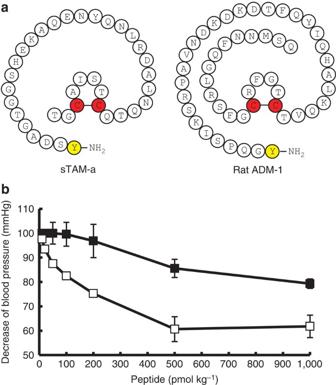Figure 2: Blood pressure-lowering activity of TAM-a. (a) Right: the predicted mature active form of TAM-a. Left: mature rat ADM-1. Red indicates the two conserved Cys residues between TAM and vertebrate ADM, and yellow indicates amidated C-terminal Tyr residues. (b) Dose-dependent blood pressure-lowering activities of sTAM-a and rat ADM-1. Standard errors of the mean (s.e.m.) were calculated based on the data sets obtained from five replicates. Open squares indicate sTAM-a and closed squares indicate rat ADM-1. Figure 2: Blood pressure-lowering activity of TAM-a. ( a ) Right: the predicted mature active form of TAM-a. Left: mature rat ADM-1. Red indicates the two conserved Cys residues between TAM and vertebrate ADM, and yellow indicates amidated C-terminal Tyr residues. ( b ) Dose-dependent blood pressure-lowering activities of sTAM-a and rat ADM-1. Standard errors of the mean (s.e.m.) were calculated based on the data sets obtained from five replicates. Open squares indicate sTAM-a and closed squares indicate rat ADM-1. Full size image HGT of vertebrate ADM into an ancestral tick A comprehensive psi-Blast analysis using all TAM isoforms as queries was performed against the NCBI database of non-redundant protein sequences, and the results showed that other invertebrates, with the exception of Ornithodoros ticks, do not have ADM-like molecules. This result was supported by similar psi-Blast analyses using vertebrate ADM-1, -2 and -5 as queries. As ADM is a specific vasoactive hormone, it is no surprise that invertebrates, which have no blood vessels, do not have ADM-like molecules. Therefore, the unique presence of TAM in Ornithodoros ticks suggests that the ADM gene might be acquired by HGT from vertebrates. To uncover the HGT signature of vertebrate ADM in Ornithodoros ticks, we analysed genomic DNA sequences encoding TAM-a and compared its exon structure with vertebrate ADM isoform exons. The exon structures of ADM-1 and ADM-2 are well conserved from fish to mammals. In addition, the ADM-5 exon structures are conserved among fish, amphibians and reptiles. However, ADM-5 is not conserved in birds and most mammals, and even the mammalian ADM-5 exon structures, which are found in few animals, are completely different from the ADM-5 exon structures in fish, amphibians and reptiles ( Supplementary Fig. 4 ). As reptiles, birds and mammals are tick host animals and if ticks actually acquired the gene encoding ADM from vertebrates, TAM might have originated from these host animals. Therefore, based on these conserved ADM exon structures and the host specificity of ticks, we selected ADM-1 and -2 from rat, that is, a mammal, and ADM-5 from a lizard, that is, a reptile, as representative examples of ADM isoforms in this analysis. The PCR-amplified genomic fragment contained two exons encoding the TAM-a molecule: the first exon encoded the secreted signal peptide sequence, and the second encoded two internal processing sites and the two key Cys residues ( Fig. 3 ). Interestingly, the second and fourth exons of ADM-1 and -5 similarly encoded the signal peptide sequence, two processing sites and the Cys residues, suggesting that the two TAM-a exons corresponded to these vertebrate ADM exons ( Fig. 3 ). TAM-a lacks the exon corresponding to the third exon of ADM-1 and -5, and because the third ADM-1 exon encodes the PAMP, TAM precursors would not be produced with a PAMP-like motif. Furthermore, a comparison of the exon nucleotide sequences between TAM-a and ADM-1 and -5 clearly showed that the exon–intron boundaries were fully conserved ( Fig. 3 and Supplementary Fig. 5 ). The second exon of TAM-a and the fourth exon of ADM-1 and -5 shared a boundary with an intron 16–22 bp upstream of the DNA sequence encoding the N-terminal processing sites. Similarly, the first exon of TAM-a and the second exon of those ADM isoforms shared a boundary with an intron 86–99 bp downstream of their initial ATG codons. Such a similarity was not observed between the exons of TAM-a and ADM-2 ( Fig. 3 and Supplementary Fig. 6 ). The third exon of ADM-2 encodes the mature molecule in a similar manner to the second exon of TAM-a, but it shares a boundary with an intron 158 bp upstream of the N-terminal processing site. Therefore, these findings suggested that TAM-a is evolutionarily close to ADM-1 and -5 but not to ADM-2 and that Ornithodoros ticks could have acquired the exons encoding vertebrate ADM-1 or -5 by HGT. 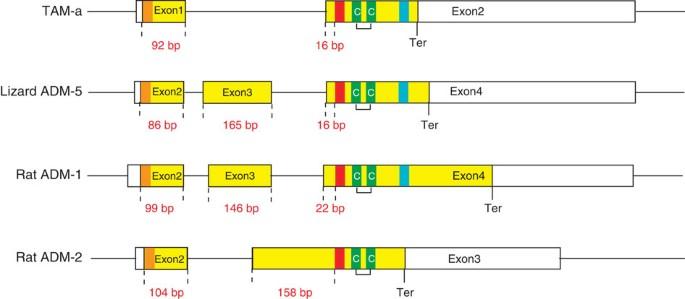Figure 3: Schematic representation of the exons and introns of TAM and major vertebrate ADMs. Genomic sequences of TAM-a (FY998678), rat (Rattus norvegicus) ADM-1 (NC_005100.3), rat ADM-2 (NC_005106.3) and lizard (Anolis carolinensis) ADM-5 (NC_014781.1) were used. Yellow indicates the regions encoding open reading frames and ‘Ter’ shows the termination codons. Red and blue show the N-terminal and C-terminal processing sites, respectively, that flank the region encoding mature ADM and TAM. In addition, orange shows the signal peptide sequences and green shows the two conserved Cys residues. Figure 3: Schematic representation of the exons and introns of TAM and major vertebrate ADMs. Genomic sequences of TAM-a (FY998678), rat ( Rattus norvegicus ) ADM-1 (NC_005100.3), rat ADM-2 (NC_005106.3) and lizard ( Anolis carolinensis ) ADM-5 (NC_014781.1) were used. Yellow indicates the regions encoding open reading frames and ‘Ter’ shows the termination codons. Red and blue show the N-terminal and C-terminal processing sites, respectively, that flank the region encoding mature ADM and TAM. In addition, orange shows the signal peptide sequences and green shows the two conserved Cys residues. Full size image In addition to the similarity among the exons, both sequence motifs of the TAM N- and C-terminal processing sites resembled those sites of ADM-1 and -5 ( Fig. 4 ). In contrast, the N-terminal processing site sequence motif of ADM-2 was vastly different from the processing site of all TAM molecules ( Fig. 4 ). Moreover, in contrast to TAM and other ADM isoforms, only ADM-2 lacked the C-terminal processing site. Therefore, these findings suggested that the sequence conservation of the processing sites correlates with exon similarity among the vertebrate ADM isoforms and TAM, providing additional evidence of the HGT of ADM-1 or -5 exons. 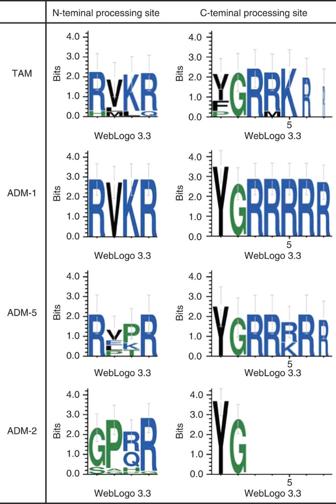Figure 4: Sequence motifs of N-terminal and C-terminal processing sites flanking the mature TAM and ADM isoforms. The sequence motifs were analysed using Weblogo version 3.3 (ref.36). As ADM-2 does not have a C-terminal processing site, the C-terminal residues of its mature form and the Gly residues that are utilized for amidation were used for motif analysis. Figure 4: Sequence motifs of N-terminal and C-terminal processing sites flanking the mature TAM and ADM isoforms. The sequence motifs were analysed using Weblogo version 3.3 (ref. 36 ). As ADM-2 does not have a C-terminal processing site, the C-terminal residues of its mature form and the Gly residues that are utilized for amidation were used for motif analysis. Full size image To further investigate the evolutionary relationship between TAM and ADM-1 and -5, we conducted a phylogenetic analysis. In this analysis, we focused on the second exon of TAM and the corresponding exons of various tetrapod ADM-1 and -5 because of the possibility that the only exon encoding the mature ADM molecule would be horizontally transmitted from a vertebrate to this tick, as discussed later. In addition, we used exons encoding mature cyclostome ADM, which were expected to be evolutionarily distant from TAM, as an out-group. Protein sequences translated from TAM and vertebrate ADM isoform exons were aligned using the ClustalW programme under the default conditions ( Supplementary Fig. 7 ). Subsequently, the phylogenetic analysis using the maximum parsimony method was performed based on the obtained sequence alignment. The resulting phylogenetic tree showed that all TAM molecules were included in the ADM-5 family ( Fig. 5 ). In contrast, the ADM-1 family and cyclostome ADM family formed distinct clusters and did not include any TAM members ( Fig. 5 ). Furthermore, we selected representative ADM-1 and -5 isoforms from vertebrates according to taxonomy and again performed the phylogenetic analysis using the maximum parsimony method. Similar results were obtained from this additional phylogenetic analysis using different sets of ADM isoforms and TAM ( Supplementary Fig. 8 ). Therefore, these results suggested that TAM might be evolutionarily closer to the vertebrate ADM-5 than to ADM-1. 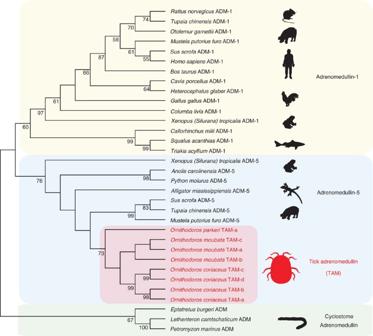Figure 5: Phylogenetic analysis of the TAM family and vertebrate ADMs. The phylogenetic tree was constructed using the maximum parsimony method based on amino acid sequences translated from the second exon of the TAM molecules and corresponding exons from various vertebrate ADMs, that is, ADM from cyclostomes and ADM-1 and -5 from chondrichthyans and tetrapods. In the resulting tree, the bootstrap values >50% are shown at each node. Figure 5: Phylogenetic analysis of the TAM family and vertebrate ADMs. The phylogenetic tree was constructed using the maximum parsimony method based on amino acid sequences translated from the second exon of the TAM molecules and corresponding exons from various vertebrate ADMs, that is, ADM from cyclostomes and ADM-1 and -5 from chondrichthyans and tetrapods. In the resulting tree, the bootstrap values >50% are shown at each node. Full size image This study suggests that the Ornithodoros tick acquired the TAM gene through the HGT of exons encoding ADM from vertebrates. The question is raised as to how the vertebrate ADM gene might have been horizontally transferred to the Ornithodoros tick. The unique biological features of ticks provide a potential explanation. In contrast to other blood-sucking arthropods, the intestinal epithelial cells of ticks engulf and ingest erythrocyte molecules and then digest them intracellularly [22] . During this process, the engulfed host molecules are released from the midgut lumen into the body cavity through transcytosis [23] . Nucleic acids present in the body cavity can rapidly diffuse within the body fluids and become incorporated into the cells of various organs [24] . Taking these features into consideration, we propose that the HGT event leading to the ancestral TAM gene acquisition occurred as follows. Host genomic DNA fragments were ingested by Ornithodoros ticks during blood-sucking and were released into the body cavity through the midgut by transcytosis. If the vertebrate hosts of ancient Ornithodoros ticks were non-mammals, as discussed later, because their erythrocytes are nucleated, genomic DNA of these erythrocytes could have been a primary source of the ancestral TAM gene. These DNA fragments could have diffused within the body cavity of the tick, reached the ovaries and entered the egg cells where genomic DNA fragments encoding ADM were accidentally integrated into the tick genome. Based on the genomic sequence analysis, the following hypotheses can be proposed to address ancestral TAM gene acquisition through HGT of the vertebrate ADM gene. The second, third and fourth exons of ADM-1 or -5 were incorporated into the Ornithodoros tick genome as a one-time event ( Fig. 3 and Supplementary Fig. 5 ), and only the third exon subsequently disappeared during evolution as it might not be necessary for vasodilation during blood feeding. The third exons of ADM-1 and -5 encode PAMP and the region between the signal peptide and N-terminal region, respectively ( Figs 1 and 3 ). Ultimately, the second and fourth exons have remained in the tick genome and are currently the two exons that constitute the ORF of TAM. Alternatively, the fourth exon of ADM-1 or -5, accompanied by part of its 5′ intron, was incorporated downstream of the 3′-end of a pre-existing exon encoding a signal peptide sequence in the tick genome. In this case, the horizontally transmitted exon of vertebrate ADM could be immediately transcribed in ticks. These two exons, the pre-existing exon and the transmitted exon, would eventually have formed the TAM gene. Given the phylogenetic analysis results, exons from ADM-5 were likely transmitted through one of the described evolutionary pathways rather than exons from ADM-1. Owing to structural and functional constraints, TAM would not be generated by natural mutations through convergent evolution. As the two conserved Cys residues and amidated C-terminal residues are required for the strict interaction between vertebrate ADM and its receptor, if any one of these essential structures is absent, the ADM vasodilatory activity is completely lost [15] . Thus, if a tick molecule acquired those essential structures in a step-by-step manner through natural mutations, evolutionary intermediates would have only a portion of those essential structures and thus would lack vasodilatory activity. Such molecules would never be selected as an ADM-like molecule, that is, TAM. These findings suggest that when Ornithodoros ticks acquired the ancestral TAM gene, the gene already encoded all these essential structures, supporting the HGT of vertebrate ADM. Furthermore, if the ancestral TAM gene evolved independently of the vertebrate ADM gene through natural mutations, TAM might not possess both N- and C-terminal processing sites; the signal peptide sequence might directly flank its mature region, and the proper C terminus might be generated by a termination codon. Therefore, the presence of two TAM processing sites suggests that the ancestral TAM gene might have already had these sites, supporting the HGT of vertebrate ADM in Ornithodoros ticks. After the HGT of vertebrate ADM into ancient ticks, the amino acid sequences of both processing sites would have been conserved under purifying selection because of functional constraints. Ticks of the Argasidae family are divided into two subfamilies, the Ornithodorinae and Argasinae subfamilies [25] ( Supplementary Fig. 9 ). Ornithodorinae subfamily ticks are further classified into five tick genera, which include the genus Ornithodoros . Molecular clock estimates regarding Argasidae family ticks place the divergence of the Ornithodorinae-Argasinae subfamilies in the Triassic period, ~234 million years ago (MYA) [26] . In addition, the fossil record of Ornithodorinae subfamily ticks suggests that ticks belonging to this subfamily had already diverged into several genera by the Cretaceous period, ~94 MYA [27] . The TAM family has been identified in all investigated Ornithodoros ticks, that is, O. moubata , O. parkeri and O. coriaceus , but it has not been detected in Argas ticks [20] , which belong to the Argasinae subfamily; however, most other salivary gland protein families, including lipocalins, Kunitz-type protease inhibitors, salivary basic tail-less proteins and putative salivary protein type-1, are conserved between these two tick subfamilies ( Supplementary Data 1 ). Therefore, these findings suggested that ancestral ticks of the genus Ornithodoros might have acquired the ADM gene by HGT from its vertebrate hosts between 234 and 94 MYA. During this period, the major terrestrial vertebrates were reptiles and dinosaurs. Reptile erythrocytes are nucleated, and dinosaur erythrocytes were deduced to possess nuclei based on the evolution of birds, which also have nucleated erythrocytes, from dinosaurs. Recently, Mans et al . [28] showed that the natural hosts of Nuttalliella namaqua , the closest living relative of ancestral ticks, are lizards, that is, reptiles. This suggests that the natural hosts of ancestral ticks might have been reptiles [28] . Thus, reptiles or dinosaurs would be expected to be the vertebrate hosts of ancestral Ornithodoros ticks, and their erythrocytes could be the origin of the TAM gene in ticks. The current vertebrate hosts of ticks of the genera Ornithodoros and Argasid are mammals and birds, respectively [29] . The haemostatic mechanisms are significantly different between mammals and birds. When blood vessels are injured in mammals, vasoconstriction and platelet aggregation immediately occur at the injury sites, triggering blood coagulation [30] , [31] . Subsequently, these three haemostatic responses enhance each other, resulting in thrombus formation. In contrast, thrombus formation rarely occurs at injury sites in birds because those three responses are less efficient than the mammalian haemostatic responses [32] . Therefore, ticks of the genus Ornithodoros prevent vasoconstriction at the feeding site on host mammals by injecting TAM and thus can overcome their haemostatic systems. If an ancient tick acquired TAM from reptiles or dinosaurs, that is, non-mammalian hosts, it might have successfully fed on blood from primitive mammals, which had already emerged during the Triassic period, by inhibiting their haemostatic system. This might have caused the expansion of its host range from ancient non-mammals to mammals. Alternatively, if an ancient tick acquired TAM from a primitive mammalian host that still retained nucleated erythrocytes, it might have coevolved and codiverged with mammalian hosts. In either case, the ancient tick that acquired TAM might have progressively become the dominant type of tick, parasitizing mammals. This tick population eventually would have become the ancestral ticks of the genus Ornithodoros . Consequently, the present study suggests that the HGT of a functional molecule might have been involved in the emergence of a new tick genus. This provides new insight into the evolution of higher eukaryotes. cDNA sequence analysis of O. moubata salivary glands Unfed female O. moubata ticks were used, which were selected to avoid contamination from host cDNA potentially present after feeding, to construct a salivary gland cDNA library. Salivary glands were dissected from tick thoraces, and poly A(+) RNA was isolated from 10 pairs of salivary glands using a QuickPrep Micro mRNA isolation kit (GE Healthcare, Waukesha, WI, USA). The salivary gland cDNA library was constructed using the SMART cDNA library construction kit according to the manufacturer’s instructions (Clontech, Palo Alto, CA, USA). One thousand cDNA clones were randomly selected, and their sequences were determined using an ABI 3100 genetic analyser (Applied Biosystems, Foster City, CA, USA). A psi-Blast analysis ( http://blast.ncbi.nlm.nih.gov/Blast.cgi ) was used to determine clonal sequence similarities, and SignalP 4.0 (ref. 33 ) was used to predict signal peptides. As salivary gland bioactive molecules are secreted into the saliva, only clones containing putative signal peptides were selected for analysis. These clones were classified into groups based on their sequence similarity. Briefly, 460 clones containing signal peptide sequences were further classified into 122 different types of molecules. Among these types, 79 were classified into six different protein families by amino acid sequence homology as described in the text. A summary of all of identified clones is presented in Supplementary Data 1 . Blood pressure-lowering activity of sTAM-a sTAM-a was synthesized using a solid phase method (Peptide Institute Inc., Japan). After synthesis, sTAM-a was purified using reverse-phase HPLC, and disulphide bond formation and C-terminal amidation were confirmed by mass spectrometry. The blood pressure-lowering activities of sTAM-a and rat ADM-1 were measured in rats. Seven-week-old male Wistar rats (280 g) were anaesthetized with an intraperitoneal injection of pentobarbital sodium (50 mg ml −1 ), and blood pressure was monitored continuously through a right femoral artery catheter (PE-50) connected to a transducer. Next, a PE-10 catheter was inserted into a vein of the left femur to administer both the maintenance solution and peptide hormones. After monitoring blood pressure for at least 60 min, sTAM-a or rat ADM-1 was injected intravenously, and changes in blood pressure were monitored for 5 min. The blood pressure-lowering activities of sTAM-a and rat ADM-1 were assessed at various concentrations ranging from 25 pmol kg −1 to 1000, pmol kg −1 . All experiments involving animals (permission number: 16-11-01) were approved by the committee of Kobe University. Cloning of genomic DNA encoding TAM-a Three female O. moubata ticks were ground in liquid nitrogen and then dissolved in TNE lysis buffer (10 mM Tris–HCl (pH 7.4), 100 mM NaCl, 25 mM EDTA and 0.5% SDS). After adding proteinase K (final concentration, 20 ng ml −1 ), the samples were incubated at 50 °C for 5 h. Genomic DNA was extracted using phenol/chloroform/isoamyl alcohol (25: 24: 1) and then precipitated with 99.5% ethanol. Purified genomic DNA was used as a template to amplify the DNA fragment encoding TAM-a with the following primers: 5′-ATGAAGTTGGCGTTCCCTGTGCTGCTAGCGC-3′ and 5′-TTATTTTTGTTTGACACTGTCCGGTAGAAGG-3′. The PCR-amplified product was cloned into the pMD20-T-vector and sequenced. TAM-a exons obtained from genomic sequences were identified by comparison with the corresponding cDNA sequences. In addition, the exons of vertebrate ADM isoforms, that is, rat ADM-1, rat ADM-2, lizard ADM-5 and pig ADM-5, were identified by comparing their genomic sequences with the cDNA sequences ( Supplementary Note 1 ). The obtained exon sequences of TAM and vertebrate ADM isoforms were utilized to compare the exon–intron boundaries of both sequences. Phylogenetic analysis of TAM and vertebrate ADM-1 and -5 Phylogenetic analyses were conducted based on sequences translated from the second exon of all TAM molecules and the corresponding exons of various vertebrate ADM-1 and -5 proteins from various vertebrates, that is, cyclostome and chondrichthyan, amphibians, reptiles, birds and mammals. As the amino acid sequences of ADM-1 are highly conserved between closely related species, for example, human and monkey, we selected representative isoforms from distantly related vertebrates to avoid redundant analyses. Genomic and cDNA sequences of ADM isoforms from selected vertebrates were collected from the NCBI database for refseq-genomic sequences and NCBI genomes. We have described this information regarding the collected genomic and cDNA sequences of vertebrate ADM in detail in Supplementary Note 1 . Next, the second exon of TAM-a and the corresponding exons of vertebrate ADM were identified by comparing the respective genomic and cDNA sequences. Five cyclostome and chondrichthyan ADM isoform exons for which genomic sequences were not available were predicted based on confirmed exon sequences of the most similar ADM isoforms ( Supplementary Note 1 ). Amino acid sequences translated from those identified exons of vertebrate ADM isoforms and all TAM molecules were aligned in the ClustalW programme built in the Mega version 5 software [34] and ‘Gonnet’ was used as a protein weight matrix. The default settings were utilized for all other conditions of amino acid sequence alignment analysis; the GAP opening penalty and GAP extension penalty were 3 and 1.8, respectively. In addition, the residue-specific penalties and hydrophobic penalties were on-state. The GAP separation distance was 4, and the end GAP separation was off-state. Subsequently, the phylogenetic tree was constructed using the maximum parsimony method based on the resulting alignment. In this analysis, we selected ‘use of all sites’ as the parameter for the Gap/Missing Data Treatment and used the default settings for all other conditions. Bootstrap tests were performed using 10,000 replicates to validate the phylogenetic relationships. Furthermore, we selected representative ADM-1 and -5 isoforms from all vertebrates according to their taxonomy, aligned those ADM isoforms and TAM by using ClustalW [35] , and then performed phylogenetic analysis using the maximum parsimony method. The conditions of alignment and phylogenetic analysis were as same as those described above. Sequence similarity and sequence alignment To investigate the distribution of ADM-like molecules, including TAM, among all living vertebrates and invertebrates, we performed psi-Blast analysis using the amino acid sequences of all TAM molecules and vertebrate ADM isoforms, as indicated in the Supplementary Note 1 . All analyses were performed against a non-redundant protein sequence database (nr) under the default conditions (expect threshold: 10; psi-blast threshold: 0.005). The amino acid sequences of all TAM molecules, which have been identified in three Ornithodoros ticks, O. moubata , O. coriaceus and O. parkeri , were aligned using the ClustalW programme [35] . According to the sequence properties of the vertebrate ADM isoforms, we predicted two processing sites, two key Cys residues and amidated C-terminal residues in the TAM molecules. Processing site sequence motif analyses in TAM and vertebrate ADM isoforms were performed using Weblogo version 3.3 (ref. 36 ). The accession numbers of all peptide hormones are detailed in Supplementary Note 1 . Accession codes: Salivary gland cDNA sequences for Ornithodoros moubata have been deposited in the GenBank expressed sequence tag (EST) database under accession codes FY998678 , FY998679 and FY998680 . How to cite this article: Iwanaga, S. et al . Horizontal gene transfer of a vertebrate vasodilatory hormone into ticks. Nat. Commun. 5:3373 doi: 10.1038/ncomms4373 (2014).